Actin remodelling factors control ciliogenesis by regulating YAP/TAZ activity and vesicle trafficking Primary cilia exert a profound impact on cell signalling and cell cycle progression. Recently, actin cytoskeleton destabilization has been recognized as a dominant inducer of ciliogenesis, but the exact mechanisms regulating ciliogenesis remain poorly understood. Here we show that the actin cytoskeleton remodelling controls ciliogenesis by regulating transcriptional coactivator YAP/TAZ as well as ciliary vesicle trafficking. Cytoplasmic retention of YAP/TAZ correlates with active ciliogenesis either in spatially confined cells or in cells treated with an actin filament destabilizer. Moreover, knockdown of YAP/TAZ is sufficient to induce ciliogenesis, whereas YAP/TAZ hyperactivation suppresses serum starvation-mediated ciliogenesis. We also identify actin remodelling factors LIMK2 and TESK1 as key players in the ciliogenesis control network in which YAP/TAZ and directional vesicle trafficking are integral components. Our work provides new insights for understanding the link between actin dynamics and ciliogenesis. Primary cilia play critical roles in transducing extracellular signals [1] , [2] and also affect the timing of cell cycle re-entry from a quiescent state [3] , [4] , [5] . Despite extensive studies that have identified many components of primary cilia/basal bodies, specific signalling pathways and transcriptional programmes governing the initiation of ciliogenesis are not well known. Withdrawal from the cell cycle is tightly associated with ciliogenesis in cultured cells, and serum starvation is a commonly used method for inducing ciliogenesis [6] , [7] , [8] . Cell confluence, eliciting contact inhibition of cell proliferation, also facilitates ciliogenesis in cultured cells [9] . However, despite the tight correlation, cell cycle exit itself is unlikely to be an absolute prerequisite for ciliogenesis in that actively cycling progenitor cells in mouse embryos display primary cilia and depend on cilium-related signalling [10] . Interestingly, recent studies have demonstrated that mechanical stimuli such as cell shape, contractility and extracellular matrix rigidity are major determinants of ciliogenic activity [11] : Cell spatial confinement, low contractility or soft extracellular substrate facilitates ciliogenesis in quiescent cells [12] . It is remarkable that actin cytoskeleton architecture is fully responsible for the regulation of ciliogenesis by these physical parameters. Several other studies have also revealed the involvement of the actin cytoskeleton in the regulation of ciliogenesis. An RNAi library screen for genes that modulate ciliogenesis identified several actin regulatory factors, including an actin-severing factor Gelsolin and an actin filament nucleator ARP2/3 complex as a positive and negative ciliogenesis regulator, respectively [13] . Moreover, an actin monomer-binding protein MIM was shown to promote ciliogenesis by antagonizing Cortactin, a nucleation-promoting factor for ARP2/3 complex [14] . A recent study also reported that a microRNA mir-129-3p promotes both ciliogenesis and cilium elongation by decreasing the expression of several actin regulatory factors that are required for branched actin network formation [15] . It is noteworthy that aberrant actin polymerization by dysregulation of Rho GTPase has been implicated in the pathogenesis of Bardet–Biedl syndrome, a model ciliopathy [16] . The organization and dynamics of the actin cytoskeleton are thought to modulate vesicular trafficking to the ciliary base and thus affect ciliary membrane biogenesis [13] , [15] . However, potential regulatory inputs from signalling cascades and nuclear factors that can mediate biological responses to actin remodelling remain largely unexplored. YAP (Yes-associated protein) and its paralogue TAZ (transcriptional coactivator with PDZ-binding motif, also known as WWTR1) are transcriptional coactivators, which interact with TEAD/TEF family of transcription factors and promote cell proliferation and survival [17] , [18] , [19] . The Hippo tumour-suppressor pathway is a key upstream regulator of YAP/TAZ, limiting their activity through phosphorylation-dependent cytoplasmic retention and destabilization. Suppression of YAP/TAZ activity by the Hippo pathway is thought to be responsible for contact inhibition of cell proliferation in cultured cells [17] , [18] . Interestingly, recent studies have shown that YAP/TAZ mediates cellular responses to mechanical cues such as cell shape and extracellular matrix rigidity [19] , [20] , [21] . Increased mechanical stresses by cell spreading or stiff extracellular substrate lead to nuclear accumulation of YAP/TAZ, whereas cell spatial confinement or soft substrate induces their cytoplasmic retention. Mechanotransduction by YAP/TAZ can operate independent of the Hippo pathway, but requires Rho GTPase and actin cytoskeletal tension [21] . Remodelling of the actin cytoskeleton by F-actin (filamentous actin)-capping or -severing proteins Cofilin (CFL), CapZ and Gelsolin appears to play an essential role in suppressing YAP/TAZ activity [20] . The remarkable similarities between cellular conditions for ciliogenesis induction and YAP/TAZ suppression prompt speculation that there might be a direct antagonistic interaction between ciliogenesis and YAP/TAZ function. Recent studies have shown that the ciliopathy proteins NPHP4 and NPHP9 negatively regulate the Hippo pathway and promote nuclear targeting of TAZ [22] , [23] . In addition, the Hippo pathway component MST1/2-SAV complex was identified as a regulator of a cilium disassembly pathway involving AURKA and HDAC6 (ref. 24 ). However, the roles of YAP/TAZ in the regulation of ciliogenesis have not been investigated in details. In this study, we demonstrate a role for YAP/TAZ in the actin cytoskeleton-dependent pathway controlling ciliogenesis, and identify key actin remodelling factors that mediate the connection between the actin cytoskeleton, YAP/TAZ and ciliogenesis. In addition, we reveal that the directional trafficking of ciliary vesicles to ciliary compartment is also controlled by the actin remodelling factors. Our results suggest that physical parameters governing ciliogenesis through actin cytoskeleton architecture may actually affect the suppression of ciliogenesis by regulating YAP/TAZ activity. Cell density affects ciliogenesis An actin filament destabilizer, cytochalasin D (CytoD), induces ciliogenesis in cultured cells [13] , serving as a useful tool for investigating actin-dependent ciliogenesis control. We first confirmed that CytoD treatment promotes ciliogenesis in human retinal pigmented epithelial (RPE1) cells ( Fig. 1a ; Supplementary Fig. 1a ). To evaluate the effect of cell density on CytoD-induced ciliogenesis, we cultured RPE1 cells either at subconfluent or confluent density and followed the time course of ciliogenesis after CytoD treatment ( Fig. 1b and Supplementary Fig. 1b ). At the subconfluent cell density, only a small subset of cells displayed primary cilia until 6 h post treatment, and thereafter ciliogenesis increased sharply. In contrast, at the higher cell density, primary cilia were already found in ∼ 45% of cells even before CytoD treatment, and ciliogenic activity reached a plateau at 6 h post treatment ( Fig. 1b ). This observation suggests that there is a cell density-dependent priming step for ciliogenesis, which takes several hours to complete. 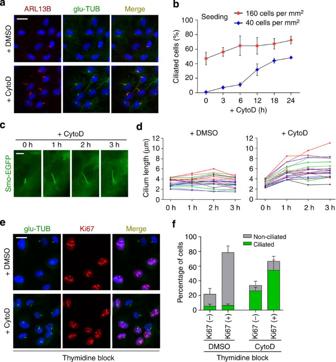Figure 1: The time course of ciliogenesis and cilium elongation induced by actin destabilization. (a) Immunofluorescence images of RPE1 cells treated with DMSO or cytochalasin D (CytoD; 200 nM) for 16 h in the presence of 10% fetal bovine serum (FBS). Cilia were double-stained with antibodies specific for poly-glutamylated Tubulin (glu-TUB) and ARL13B. Blue channel was used for 4,6-diamidino-2-phenylindole (DAPI) staining. (b) Line graph of ciliated cell frequency in RPE1 cells plated in two different densities and treated with CytoD for the indicated times. Seeding density: 40 cells per mm2(low density), 160 cells per mm2(high density). See alsoSupplementary Fig. 1b. Error bars are s.e.m. (n=3 independent experiments). (c) Time-lapse imaging of a live RPE1 cell stably expressing Smo-EGFP (RPE1-Smo-EGFP) for up to 3 h after CytoD treatment. (d) Graph showing the changes of ciliary length of RPE1-Smo-EGFP cell treated with DMSO or CytoD from time-lapse microscopic images (n=20 cells for each treatment). Smo-EGFP fluorescence was used for the measurement of cilium length. (e) Immunofluorescence images of RPE1 cells treated with DMSO or CytoD for 18 h in the early S phase arrest with a single thymidine block (36 h before fixation). Cilia were stained with anti-glu-TUB antibody. (f) Quantification of experiments illustrated ine. Error bars are s.d. (n=2 independent experiments). Scale bars ina,eare 20 μm, andcis 5 μm. Figure 1: The time course of ciliogenesis and cilium elongation induced by actin destabilization. ( a ) Immunofluorescence images of RPE1 cells treated with DMSO or cytochalasin D (CytoD; 200 nM) for 16 h in the presence of 10% fetal bovine serum (FBS). Cilia were double-stained with antibodies specific for poly-glutamylated Tubulin (glu-TUB) and ARL13B. Blue channel was used for 4,6-diamidino-2-phenylindole (DAPI) staining. ( b ) Line graph of ciliated cell frequency in RPE1 cells plated in two different densities and treated with CytoD for the indicated times. Seeding density: 40 cells per mm 2 (low density), 160 cells per mm 2 (high density). See also Supplementary Fig. 1b . Error bars are s.e.m. ( n =3 independent experiments). ( c ) Time-lapse imaging of a live RPE1 cell stably expressing Smo-EGFP (RPE1-Smo-EGFP) for up to 3 h after CytoD treatment. ( d ) Graph showing the changes of ciliary length of RPE1-Smo-EGFP cell treated with DMSO or CytoD from time-lapse microscopic images ( n =20 cells for each treatment). Smo-EGFP fluorescence was used for the measurement of cilium length. ( e ) Immunofluorescence images of RPE1 cells treated with DMSO or CytoD for 18 h in the early S phase arrest with a single thymidine block (36 h before fixation). Cilia were stained with anti-glu-TUB antibody. ( f ) Quantification of experiments illustrated in e . Error bars are s.d. ( n =2 independent experiments). Scale bars in a , e are 20 μm, and c is 5 μm. Full size image In addition to inducing ciliogenesis, CytoD promotes the elongation of pre-existing cilia ( Fig. 1c,d ). We imaged live RPE1 cells stably expressing EGFP-tagged Smoothened (Smo-EGFP), which is a transmembrane protein specifically targeted to the ciliary membrane. Cilium elongation mainly occurred at the first hour after treatment and the elongation rate decreased thereafter even in the presence of CytoD (0–1 h, 2.24±0.19 μm h −1 ; 1–2 h, 0.44±0.22 μm h −1 ; 2–3 h, 0.16±0.12 μm h −1 (mean±s.e.m., n =20 cells)). As reported previously [13] , CytoD treatment changed the distribution of Smo-EGFP ( Supplementary Fig. 1c ). CytoD increased the number of discrete Smo-EGFP-positive vesicles around the centrosome as well as in the cytoplasm in less than 1 h. Moreover, the small GTPases RAB8 and RAB11, which are known to function in membrane trafficking to the ciliary base [25] , [26] , were redistributed to the centrosomal area in response to CytoD treatment within 1 or 2 h ( Supplementary Fig. 1c ). Thus, both cilium elongation and reorganization of vesicle trafficking are unlikely to be rate-limiting processes in the progression of CytoD-induced ciliogenesis. Next, we asked whether ciliogenesis occurs in a delayed manner at subconfluent cell densities because cell cycle quiescence or exit must precede the assembly of cilia. Indeed, CytoD-induced ciliogenesis was accompanied by a substantial decrease in the number of RPE1 cells expressing Ki67, a marker for cellular proliferation ( Supplementary Fig. 2a ). However, this observation does not exclude the possibility that cell cycle quiescence and ciliogenesis are processes running in parallel without direct causality. To address this, we arrested cells in early S phase by a thymidine block, and then treated them with CytoD. Remarkably, CytoD triggered ciliogenesis in both Ki67-negative G0 phase cells and Ki67-positive interphase cells ( Fig. 1e,f ). In addition, CytoD efficiently induced ciliogenesis in cells arrested in G2 phase as a consequence of DNA damage by γ-irradiation ( Supplementary Fig. 2b–d ). These results suggest that cell cycle quiescence is not a prerequisite for cilium assembly in RPE1 cells at least in the presence of CytoD. Cytoplasmic retention of YAP/TAZ correlates with ciliogenesis YAP and TAZ are potent transcriptional coactivators for TEAD/TEF family of transcription factors. Cytoplasmic relocalization of YAP/TAZ, which inactivates them, has been shown to occur in response to actin depolymerization or increased cell–cell contact [21] , [27] , [28] . We confirmed that cell density affects YAP/TAZ localization in RPE1 cells ( Supplementary Fig. 3a ), and then examined potential correlation between YAP/TAZ localization and ciliogenesis. As shown in Fig. 2a , in most areas of lower cell densities, nuclear YAP/TAZ enrichment was apparent and cilia were not found. In contrast, ciliated cells were mainly found in areas of higher cell densities where YAP/TAZ were retained in the cytoplasm. Moreover, CytoD treatment caused both the relocalization of YAP/TAZ from the nucleus to the cytoplasm and the assembly of primary cilia even in subconfluent culture ( Fig. 2b ). Similar patterns were observed in cells arrested in early S phase, suggesting that the correlation is independent of the roles of YAP/TAZ in cell proliferation ( Supplementary Fig. 3b ). To further evaluate the correlation, we measured YAP/TAZ fluorescence intensities from the nucleus and the cytoplasm. Then, we calculated the nuclear/cytoplasmic fluorescence intensity ratio (N/C ratio) of YAP/TAZ, and defined YAP/TAZ distribution patterns either as nuclear (N/C ratio>1.2) or non-nuclear (N/C ratio≤1.2; see Supplementary Fig. 3c for details). The proportion of cells forming cilia in response to CytoD was significantly higher among cells exhibiting non-nuclear YAP/TAZ when compared with cells exhibiting nuclear YAP/TAZ (non-nuclear, 35.3%; nuclear, 18.1% ( n =3 independent experiments; unpaired Student t -test, P <0.05); Fig. 2c ). Thus, YAP/TAZ activity is inversely correlated with cellular ciliogenic potential. 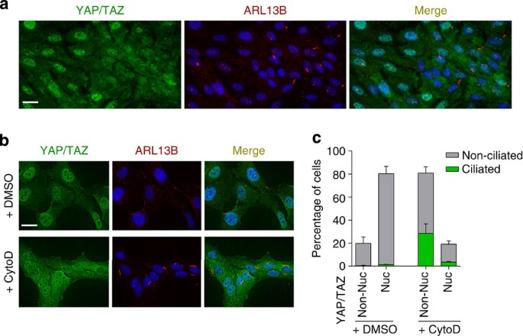Figure 2: Cytoplasmic retention of YAP/TAZ correlates with cilium formation. (a) Immunofluorescence images displaying the difference of YAP/TAZ subcellular localization and ciliogenesis according to the local cell density. RPE1 cells were cultured in media with 10% FBS until they reach confluence. An antibody detecting both YAP and TAZ was used. (b) Cytoplasmic sequestration of YAP/TAZ and concurrent induction of ciliogenesis in cells treated with CytoD for 12 h in the presence of 10% FBS. (c) Quantification of experiments illustrated inb. Cells were classified either as Nuclear (Nuc) if the nuclear/cytoplasmic fluorescence intensity ratio of YAP/TAZ is greater than 1.2 or non-Nuclear (non-Nuc) if not. SeeSupplementary Fig. 3cfor details. Error bars are s.d. (n=3 independent experiments). All scale bars are 20 μm. Figure 2: Cytoplasmic retention of YAP/TAZ correlates with cilium formation. ( a ) Immunofluorescence images displaying the difference of YAP/TAZ subcellular localization and ciliogenesis according to the local cell density. RPE1 cells were cultured in media with 10% FBS until they reach confluence. An antibody detecting both YAP and TAZ was used. ( b ) Cytoplasmic sequestration of YAP/TAZ and concurrent induction of ciliogenesis in cells treated with CytoD for 12 h in the presence of 10% FBS. ( c ) Quantification of experiments illustrated in b . Cells were classified either as Nuclear (Nuc) if the nuclear/cytoplasmic fluorescence intensity ratio of YAP/TAZ is greater than 1.2 or non-Nuclear (non-Nuc) if not. See Supplementary Fig. 3c for details. Error bars are s.d. ( n =3 independent experiments). All scale bars are 20 μm. Full size image Lysophosphatidic acid (LPA) is a glycerophospholipid signalling molecule abundant in serum and acts through specific G-protein-coupled receptors [29] . Recent studies have shown that LPA activates YAP/TAZ through modulation of Rho GTPase activity and the actin cytoskeleton [30] . Therefore, we tested if activation of YAP/TAZ by LPA can suppress the assembly of primary cilia. As expected, LPA treatment facilitated both actin filament assembly and nuclear shift of YAP/TAZ localization in cells cultured at confluence in serum-free media ( Fig. 3a and Supplementary Fig. 4a ). Remarkably, nuclear YAP/TAZ accumulation was accompanied by suppression of serum starvation-mediated ciliogenesis ( Fig. 3a,b ). Cilium length was also decreased by LPA treatment in a dose-dependent manner ( Fig. 3b ). These results suggest that actin cytoskeleton plays a dominant role in suppressing cilium assembly, possibly through YAP/TAZ activation. 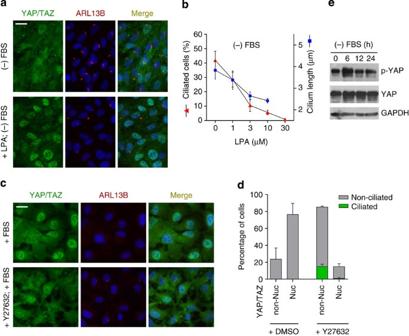Figure 3: Modulation of YAP/TAZ activity is accompanied by changes in ciliogenic activity. (a) Immunofluorescence images showing the nuclear enrichment of YAP/TAZ and concurrent inhibition of ciliogenesis by lysophosphatidic acid (LPA; 10 μM) treatment (24 h) in RPE1 cells, which were serum starved for 24 h. (b) Line graph showing the suppression of ciliogenesis and cilium elongation by LPA treatment. Confluent cells were serum-starved for 24 h with or without LPA treatment at the indicated concentrations. (c) Immunoblot analyses for YAP and phospho-YAP (Ser127) in cells, which were harvested in subconfluence at the indicated times after serum removal. Glyceraldehyde 3-phosphate dehydrogenase (GAPDH) was used as a loading control. (d) Subconfluent (50–75%) RPE1 cells were treated with a ROCK inhibitor, Y27632 (25 μM) for 24 h in the presence of 10% FBS. (e) Quantification of experiments illustrated ind. All error bars are s.d. (n=3 independent experiments). All scale bars are 20 μm. Figure 3: Modulation of YAP/TAZ activity is accompanied by changes in ciliogenic activity. ( a ) Immunofluorescence images showing the nuclear enrichment of YAP/TAZ and concurrent inhibition of ciliogenesis by lysophosphatidic acid (LPA; 10 μM) treatment (24 h) in RPE1 cells, which were serum starved for 24 h. ( b ) Line graph showing the suppression of ciliogenesis and cilium elongation by LPA treatment. Confluent cells were serum-starved for 24 h with or without LPA treatment at the indicated concentrations. ( c ) Immunoblot analyses for YAP and phospho-YAP (Ser127) in cells, which were harvested in subconfluence at the indicated times after serum removal. Glyceraldehyde 3-phosphate dehydrogenase (GAPDH) was used as a loading control. ( d ) Subconfluent (50–75%) RPE1 cells were treated with a ROCK inhibitor, Y27632 (25 μM) for 24 h in the presence of 10% FBS. ( e ) Quantification of experiments illustrated in d . All error bars are s.d. ( n =3 independent experiments). All scale bars are 20 μm. Full size image Because the Rho GTPase pathway is involved in the control of YAP/TAZ [30] as well as actin dynamics, we examined the effect of Rho kinase (ROCK) inhibitor, Y27362. RPE1 cells treated with Y27362 exhibited cytoplasmic retention of YAP/TAZ as well as a dramatic reorganization of the actin cytoskeleton ( Fig. 3c and Supplementary Fig. 4b ). In accordance with this, our fluorescence resonance energy transfer (FRET)-based analysis demonstrated that cells exhibiting cytoplasmic YAP/TAZ retention display relatively low levels of RhoA activity ( Supplementary Fig. 4c,d ). Crucially, Y27362 promoted ciliogenesis preferentially in cells in which YAP/TAZ were retained in the cytoplasm ( Fig. 3d ), confirming that YAP/TAZ is intimately associate with ciliogenesis. We next tested if serum starvation, which promotes ciliogenesis, affects YAP/TAZ activity. YAP phosphorylation is known to block YAP nuclear enrichment [17] , [18] . As shown in Fig. 3e , we observed an increase in phospho-YAP level at 6 h post-serum removal, and then phospho-YAP returned to basal levels. It is likely that a decrease in YAP/TAZ activity due to the absence of serum-borne LPA is a contributing factor for serum starvation-mediated ciliogenesis. Next, we tested if cell culture density, which is a critical determinant of both YAP/TAZ and ciliogenic activity, affects the actin cytoskeletal organization in RPE1 cells. Previously, it was shown that RPE1 cells display larger stress fibres as the degree of cell spreading increases [12] . Cell spreading is limited in higher cell densities and as shown in Supplementary Fig. 4e , the number and size of stress fibres was slightly decreased in cells maintained at confluence for 24 h. Instead, we observed a prominent increase in the number and size of non-filamentous actin aggregates. Similarly, CytoD treatment also disrupted actin fibres and promoted the formation of non-filamentous actin aggregates ( Supplementary Fig. 4e ). Together, these observations further support the functional link between actin dynamics, YAP/TAZ and ciliogenesis. YAP/TAZ upregulates negative ciliogenesis regulators To investigate the role of YAP/TAZ in the negative regulation of ciliogenesis, we performed small interfering RNA (siRNA)-mediated knockdown experiments. Remarkably, knockdown of either YAP or TAZ caused an increase in the number of ciliated cells in the absence of serum starvation ( Fig. 4a,b ). TAZ knockdown was more efficient in inducing ciliogenesis than YAP knockdown. YAP/TAZ double-knockdown further enhanced ciliogenesis, suggesting a certain degree of functional redundancy. As shown in Fig. 4c , LPA failed to suppress serum starvation-mediated ciliogenesis in cells co-transfected with YAP/TAZ mix siRNAs. This result confirms that YAP/TAZ activation indeed mediates the inhibitory effect of LPA on ciliogenesis. The involvement of YAP/TAZ in the negative regulation of ciliogenesis was also demonstrated in a cancer cell line A549 ( Supplementary Fig. 5a–c ). To further confirm anti-ciliogenic potential of YAP, we transiently overexpressed YAP-5SA, a hyperactive YAP mutant in which all five inactivating phosphorylation sites were eliminated [31] . As shown in Fig. 4d , serum starvation-mediated ciliogenesis was significantly inhibited by YAP-5SA, whereas overexpression of a TEAD-binding defective YAP mutant [32] (YAP-5SA-S94A) was not efficient in suppressing ciliogenesis. Taken together, these results indicate that YAP/TAZ plays a role in the negative regulation of ciliogenesis. Centriole migration to the apical plasma membrane is one of the first steps of ciliogenesis. YAP-5SA overexpression did not affect the position of the centrioles along z axis in serum-starved cells ( Supplementary Fig. 6a ), suggesting that centriole migration is independent of YAP activity in RPE1 cells. 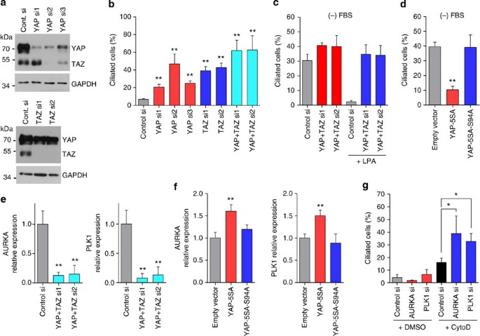Figure 4: YAP/TAZ inhibit ciliogenesis and upregulate the expression of AURKA and PLK1. (a) Immunoblotting to confirm siRNA-mediated knockdown of YAP and TAZ. RPE1 cells were transfected with the indicated siRNAs for 60 h. Transfection of YAP si2 depleted both YAP and TAZ. Glyceraldehyde 3-phosphate dehydrogenase (GAPDH) was used as a loading control. (b) Quantification of ciliogenesis in cells transfected with YAP, TAZ and YAP/TAZ mix siRNAs for 60 h in the presence of 10% FBS. (c) Graph of ciliated cell frequency in cells co-depleted with YAP and TAZ in the absence of serum. LPA (30 μM) was added to the culture media 24 h before fixation. (d) Quantification of ciliogenesis in cells infected with retroviruses carrying an empty vector, YAP-5SA (a hyperactive YAP mutant) or YAP-5SA-S94A (a hyperactive YAP mutant without TEAD-binding capacity), and then cultured in serum-free media for 48 h. (e) Quantitative RT–PCR (qRT–PCR) analyses of the expression ofAURKAandPLK1in cells transfected with YAP/TAZ mix siRNAs for 60 h.GAPDHwas used as a normalization control. (f) qRT–PCR analyses of the expression ofAURKAandPLK1in cells infected with retroviruses carrying an empty vector, YAP-5SA or YAP-5SA-S94A, and then cultured in the presence of serum for 48 h. (g) Graph showing the ciliated cell percentage in cells transfected with the AURKA and PLK1 siRNAs for 60 h. DMSO or CytoD was added to the culture media 6 h before fixation. All error bars are s.d. (n=3 independent experiments). TheP-values were determined by unpaired Student’st-test; *P<0.05, **P<0.01. Figure 4: YAP/TAZ inhibit ciliogenesis and upregulate the expression of AURKA and PLK1. ( a ) Immunoblotting to confirm siRNA-mediated knockdown of YAP and TAZ. RPE1 cells were transfected with the indicated siRNAs for 60 h. Transfection of YAP si2 depleted both YAP and TAZ. Glyceraldehyde 3-phosphate dehydrogenase (GAPDH) was used as a loading control. ( b ) Quantification of ciliogenesis in cells transfected with YAP, TAZ and YAP/TAZ mix siRNAs for 60 h in the presence of 10% FBS. ( c ) Graph of ciliated cell frequency in cells co-depleted with YAP and TAZ in the absence of serum. LPA (30 μM) was added to the culture media 24 h before fixation. ( d ) Quantification of ciliogenesis in cells infected with retroviruses carrying an empty vector, YAP-5SA (a hyperactive YAP mutant) or YAP-5SA-S94A (a hyperactive YAP mutant without TEAD-binding capacity), and then cultured in serum-free media for 48 h. ( e ) Quantitative RT–PCR (qRT–PCR) analyses of the expression of AURKA and PLK1 in cells transfected with YAP/TAZ mix siRNAs for 60 h. GAPDH was used as a normalization control. ( f ) qRT–PCR analyses of the expression of AURKA and PLK1 in cells infected with retroviruses carrying an empty vector, YAP-5SA or YAP-5SA-S94A, and then cultured in the presence of serum for 48 h. ( g ) Graph showing the ciliated cell percentage in cells transfected with the AURKA and PLK1 siRNAs for 60 h. DMSO or CytoD was added to the culture media 6 h before fixation. All error bars are s.d. ( n =3 independent experiments). The P -values were determined by unpaired Student’s t -test; * P <0.05, ** P <0.01. Full size image To gain mechanistic insight into the link between YAP/TAZ and ciliogenesis, we asked if there are target genes of YAP/TAZ, which are known to control ciliogenesis. We reviewed the literatures that reported YAP/TAZ target genes by using microarray gene expression analyses [32] , [33] . Interestingly, genes whose expression is repeatedly correlated with YAP activity includes Aurora A kinase ( AURKA ) and Polo-like kinase 1 ( PLK1 ), which are known to mediate cilium disassembly [5] , [34] and ciliogenesis inhibition [35] . In addition, Encyclopedia of DNA elements-chromatin immunoprecipitation with massively parallel DNA sequencing data reveal the binding of TEAD4 in the promoter region of both AURKA and PLK1 genes [36] . Thus, we tested whether YAP/TAZ control the expression of AURKA and PLK1 in RPE1 cells. As expected, our quantitative reverse transcription–PCR (qRT–PCR) analyses confirmed that the expression levels of both AURKA and PLK1 decreased in cells depleted of YAP/TAZ ( Fig. 4e ). Moreover, overexpression of YAP-5SA enhanced the expression of AURKA and PLK1 ( Fig. 4f ). Next, we asked if suppression of the expression of either AURKA or PLK1 is sufficient to trigger ciliogenesis in the absence of other ciliogenic stimulations. Although siRNAs that we used efficiently depleted AURKA and PLK1 transcripts ( Supplementary Fig. 6b ), active ciliogenesis was not observed in cells transfected with the siRNAs ( Fig. 4g ). However, the proportion of cells developing cilia at an early time point after CytoD treatment increased significantly after AURKA or PLK1 knockdown ( Fig. 4g ). It is possible that degradation of pre-existing AURKA and PLK1 transcripts or proteins occurring after YAP/TAZ cytoplasmic sequestration contributes to the delay in CytoD-induced ciliogenesis ( Fig. 1b ). We then examined the requirement for new protein synthesis during ciliogenesis, using a protein synthesis inhibitor, cycloheximide (CHX). CHX did not exert any ciliogenic effect ( Supplementary Fig. 6c,d ). Besides, CHX treatment blocked the ciliogenic effect of CytoD or serum starvation. These results indicate that ciliogenesis depends not only on the suppression of negative regulators but also on upregulation of either positive regulators or essential ciliary components. The Hippo pathway is known as the major upstream regulator of YAP/TAZ activity [17] , [18] . Hippo pathway components LATS1/2 kinases phosphorylate and inhibit nuclear targeting of YAP/TAZ. Therefore, we tested whether Hippo pathway activation is involved in ciliogenesis through its role in YAP/TAZ inhibition. Unexpectedly, LATS1 and LATS2 knockdown did not decrease the number of ciliated cells in a serum-starvation condition ( Fig. 5a,b ). Elevation of YAP/TAZ activities in LATS1/2-depleted cells was confirmed by both the increase in the proportion of cells exhibiting nuclear YAP/TAZ enrichment ( Fig. 5c ) and the upregulation of AURKA and PLK1 expression ( Fig. 5d,e ). However, it should be noted that the levels of AURKA and PLK1 in LATS1/2-depleted cells in the serum-starvation condition is significantly lower than those in controls cells cultured in the presence of 10% FBS. Thus, it is likely that YAP/TAZ activation induced by LATS1/2 depletion was insufficient to inhibit ciliogenesis in a serum-starvation condition. Recent studies have demonstrated that physical/mechanical stimuli, which affect Rho activity and actin cytoskeletal tension, can control YAP/TAZ activity in a Hippo pathway-independent manner [21] . Thus, it is possible that Hippo-independent mechanisms also play a role in suppressing YAP/TAZ activity during the progression of serum starvation-mediated ciliogenesis. 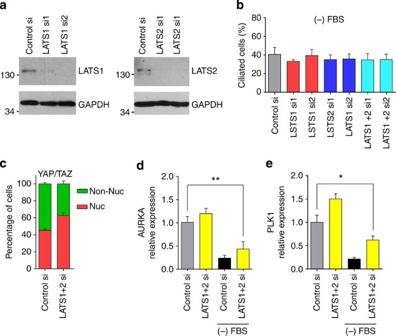Figure 5: LATS1/2 is dispensable for serum starvation-mediated ciliogenesis. (a) Immunoblotting to confirm siRNA-mediated knockdown of LATS1 and LATS2. RPE1 cells were transfected with the indicated siRNAs for 72 h. (b) Quantification of ciliogenesis in cells transfected with the LATS1, LATS2 and LATS1/2 mix siRNAs for 72 h. Cells were serum-starved for 24 h before fixation. (c) Quantification of the subcellular localization of YAP/TAZ in cells double-transfected with LATS1 and LATS2 siRNAs. (d,e) qRT–PCR analyses of the expression ofAURKAandPLK1in cells co-transfected with LATS1 and LATS2 siRNAs.GAPDHwas used as a normalization control. All error bars are s.d. (n=3 independent experiments). TheP-values were determined by unpaired Student’st-test; *P<0.05, **P<0.01. Figure 5: LATS1/2 is dispensable for serum starvation-mediated ciliogenesis. ( a ) Immunoblotting to confirm siRNA-mediated knockdown of LATS1 and LATS2. RPE1 cells were transfected with the indicated siRNAs for 72 h. ( b ) Quantification of ciliogenesis in cells transfected with the LATS1, LATS2 and LATS1/2 mix siRNAs for 72 h. Cells were serum-starved for 24 h before fixation. ( c ) Quantification of the subcellular localization of YAP/TAZ in cells double-transfected with LATS1 and LATS2 siRNAs. ( d , e ) qRT–PCR analyses of the expression of AURKA and PLK1 in cells co-transfected with LATS1 and LATS2 siRNAs. GAPDH was used as a normalization control. All error bars are s.d. ( n =3 independent experiments). The P -values were determined by unpaired Student’s t -test; * P <0.05, ** P <0.01. Full size image LIMK2 and TESK1 control CFL to suppress ciliogenesis Data presented so far suggest that the experimental perturbation of actin filament architecture affects ciliogenesis through YAP/TAZ regulation. Next, we sought to identify actin cytoskeleton remodelling factors, which modulate ciliogenic activity as upstream regulators of YAP/TAZ. We focused on kinases controlling actin dynamics and performed a siRNA-based screen. RPE1 cells were transfected with pooled siRNAs targeting 13 actin regulatory kinases, and cilium formation in response to serum starvation was assessed. As shown in Fig. 6a , depletion of several kinases increased the percentage of ciliated cells relative to control, and two top candidates LIM kinase 2 (LIMK2) and testicular protein kinase 1 (TESK1) were selected for further studies. Both LIMK2 and TESK1 are serine/threonine kinases, which are known to inactivate the actin-severing protein CFL via phosphorylation at serine 3 (ref. 37 ). To confirm that knockdown of these candidates is sufficient for inducing ciliogenesis, we transfected cells with two distinct siRNAs and ciliogenesis was monitored in the absence of other ciliogenic stimulations. Depletion of LIMK2 and TESK1 was confirmed by immunoblotting and qRT–PCR, respectively ( Fig. 6b,c ). Notably, knockdown of either LIMK2 or TESK1 significantly increased the number of ciliated cells, suggesting that LIMK2 and TESK1 play a role in the negative regulation of ciliogenesis ( Fig. 6d ). Involvement of TESK1 in the suppression of ciliogenesis was further supported by the observation that TESK1 overexpression interferes with serum starvation-mediated ciliogenesis ( Fig. 6e ). 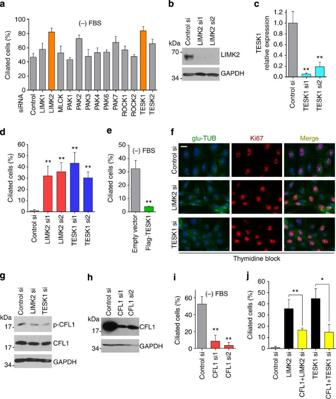Figure 6: Actin remodelling factors LIMK2 and TESK1 repress ciliogenesis. (a) Quantification of ciliogenesis in RPE1 cells transfected with pooled siRNAs targeting kinases involved in actin dynamics for 72 h. Cells were serum-starved for final 48 h. (b) Immunoblotting to confirm siRNA-mediated knockdown of LIMK2. Glyceraldehyde 3-phosphate dehydrogenase (GAPDH) was used as a loading control. (c) qRT–PCR to confirm siRNA-mediated depletion ofTESK1transcripts.GAPDHwas used as a normalization control. (d) Quantification of ciliogenesis in cells transfected with LIMK2 and TESK1 siRNAs for 72 h without serum starvation. (e) Quantification of ciliated cell frequency in cells transfected with flag-tagged TESK1 vector. Cells were serum-starved for final 24 h. (f) Immunofluorescence image displaying the effect of LIMK2 and TESK1 knockdown on ciliogenesis in cells arrested in early S phase using a single thymidine block for 36 h before fixation. Scale bar is 20 μm. (g) Immunoblot analyses of CFL and phospho-CFL after LIMK2 or TESK1 knockdown. GAPDH was used as a loading control. (h) Immunoblotting to confirm siRNA-mediated knockdown of CFL. GAPDH was used as a loading control. (i) Quantification of ciliogenesis in cells depleted with CFL and serum-starved for 24 h. (j) Quantification of ciliated cell percentage in cells transfected with indicated siRNAs without serum starvation. All error bars are s.d. (a,c,n=2;d,e,i,j,n=3 independent experiments). TheP-values were determined by unpaired Student’st-test; *P<0.05, **P<0.01. Figure 6: Actin remodelling factors LIMK2 and TESK1 repress ciliogenesis. ( a ) Quantification of ciliogenesis in RPE1 cells transfected with pooled siRNAs targeting kinases involved in actin dynamics for 72 h. Cells were serum-starved for final 48 h. ( b ) Immunoblotting to confirm siRNA-mediated knockdown of LIMK2. Glyceraldehyde 3-phosphate dehydrogenase (GAPDH) was used as a loading control. ( c ) qRT–PCR to confirm siRNA-mediated depletion of TESK1 transcripts. GAPDH was used as a normalization control. ( d ) Quantification of ciliogenesis in cells transfected with LIMK2 and TESK1 siRNAs for 72 h without serum starvation. ( e ) Quantification of ciliated cell frequency in cells transfected with flag-tagged TESK1 vector. Cells were serum-starved for final 24 h. ( f ) Immunofluorescence image displaying the effect of LIMK2 and TESK1 knockdown on ciliogenesis in cells arrested in early S phase using a single thymidine block for 36 h before fixation. Scale bar is 20 μm. ( g ) Immunoblot analyses of CFL and phospho-CFL after LIMK2 or TESK1 knockdown. GAPDH was used as a loading control. ( h ) Immunoblotting to confirm siRNA-mediated knockdown of CFL. GAPDH was used as a loading control. ( i ) Quantification of ciliogenesis in cells depleted with CFL and serum-starved for 24 h. ( j ) Quantification of ciliated cell percentage in cells transfected with indicated siRNAs without serum starvation. All error bars are s.d. ( a , c , n =2; d , e , i , j , n =3 independent experiments). The P -values were determined by unpaired Student’s t -test; * P <0.05, ** P <0.01. Full size image We also examined the changes in the actin cytoskeleton after LIMK2 and TESK1 knockdown. As shown in Supplementary Fig. 7a , the number and size of stress fibres decreased in LIMK2-depleted cells, whereas cellular edge areas displayed prominent accumulations of actin filaments. In TESK1-depleted cells, large stress fibres are rarely observed, whereas thinner actin filaments were arranged radially. In addition, the cortical actin at the central area became more pronounced in TESK1-depleted cells ( Supplementary Fig. 7b ). The knockdown of either LIMK2 or TESK1 resulted in a substantial decrease in the number of Ki67-positive cells in the presence of serum ( Supplementary Fig. 7c ). However, similar to CytoD effect ( Fig. 1e,f ), LIMK2 or TESK1 knockdown caused an induction of ciliogenesis even in cells arrested in early S phase by a thymidine block ( Fig. 6f ). These observations suggest that LIMK2 and TESK1 affect ciliogenesis through their roles in the actin cytoskeleton remodelling. Because LIMK2 and TESK1 are known to control actin dynamics through CFL, we investigated the involvement of CFL in the regulation of ciliogenesis. First, the phosphorylation levels of Cofilin1 (CFL1), a non-muscle isoform of Cofilin, decreased in response to the knockdown of either LIMK2 or TESK1 ( Fig. 6g and Supplementary Fig. 7d,e ). Second, serum starvation-mediated ciliogenesis was efficiently suppressed by the depletion of CFL1, demonstrating positive roles of CFL1 in ciliogenesis ( Fig. 6h,i ). Moreover, the increase in ciliogenic activities in LIMK2- or TESK1-depleted cells was significantly suppressed by double-knockdown with CFL1 ( Fig. 6j ). These results indicate that CFL1 activation underlies the promotion of ciliogenesis in response to LIMK2 or TESK1 depletion. LIMK2 and TESK1 promote YAP/TAZ activity We next asked whether actin cytoskeleton remodelling orchestrated by LIMK2/TESK1-CFL axis affects ciliogenesis through the modulation of YAP/TAZ activity. To address this question, we first examined the effect of LIMK2 and TESK1 knockdown on the distribution of YAP/TAZ. As shown in Fig. 7a , cells depleted of either LIMK2 or TESK1 displayed cytoplasmic retention of YAP/TAZ at subconfluence. We also performed luciferase assay, using a YAP/TAZ-responsive reporter (8xGTIIC-luciferase), which contains eight TEAD-binding sites [21] . Crucially, YAP/TAZ relocalization in LIMK2/TESK1-depleted cells was paralleled by a significant suppression of the reporter activity ( Fig. 7b ). We then tested the effect of LIMKi3, a LIMK1/2-specific inhibitor blocking the kinase activity [38] . LIMKi3 treatment induced redistribution of YAP/TAZ from nucleus to cytoplasm in a subset of cells in a dose-dependent manner ( Fig. 7c ). In addition, as expected, LIMKi3-mediated cytoplasmic retention of YAP/TAZ was accompanied by an induction of ciliogenesis ( Fig. 7d and Supplementary Fig. 8a ). Collectively, these data suggest that LIMK2 and TESK1 control ciliogenesis by modulating YAP/TAZ activity. 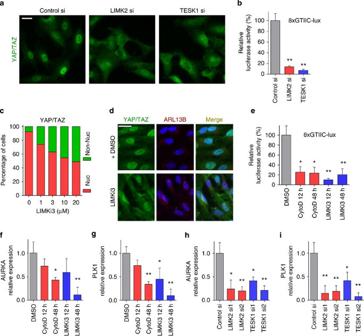Figure 7: LIMK2 and TESK1 affect both the activity of YAP/TAZ and the expression of AURKA and PLK1. (a) Immunofluorescence images of subconfluent RPE1 cells transfected with LIMK2 and TESK1 siRNAs for 48 h. (b) Luciferase assay with the YAP/TAZ-responsive reporter, 8xGTIIC-luciferase (8xGTIIC-lux) in cells transfected with the indicated siRNAs for 48 h. Luciferase activity was normalized by β-galactosidase activity. (c) Quantification of YAP/TAZ immunolocalization in cells treated with LIMKi3 (LIMK1/2 inhibitor) at the indicated concentrations for 6 h (n=100 cells for each condition). (d) Immunofluorescence images of cells treated with LIMKi3 (20 μM) for 24 h. (e) Luciferase assay with YAP/TAZ-responsive reporter 8xGTIIC-lux in cells treated with CytoD or LIMKi3 for 24 and 48 h. Luciferase activity was normalized by β-galactosidase activity. (f,g) qRT–PCR analyses of the expression ofAURKAandPLK1in cells treated with CytoD or LIMKi3 for 24 and 48 h.GAPDHwas used as a normalization control. (h,i) qRT–PCR analyses of the expression ofAURKAandPLK1in cells transfected with the indicated siRNAs for 60 h. All scale bars are 20 μm. All error bars are s.d. (n=3 independent experiments). TheP-values were determined by unpaired Student’st-test; *P<0.05, **P<0.01. Figure 7: LIMK2 and TESK1 affect both the activity of YAP/TAZ and the expression of AURKA and PLK1. ( a ) Immunofluorescence images of subconfluent RPE1 cells transfected with LIMK2 and TESK1 siRNAs for 48 h. ( b ) Luciferase assay with the YAP/TAZ-responsive reporter, 8xGTIIC-luciferase (8xGTIIC-lux) in cells transfected with the indicated siRNAs for 48 h. Luciferase activity was normalized by β-galactosidase activity. ( c ) Quantification of YAP/TAZ immunolocalization in cells treated with LIMKi3 (LIMK1/2 inhibitor) at the indicated concentrations for 6 h ( n =100 cells for each condition). ( d ) Immunofluorescence images of cells treated with LIMKi3 (20 μM) for 24 h. ( e ) Luciferase assay with YAP/TAZ-responsive reporter 8xGTIIC-lux in cells treated with CytoD or LIMKi3 for 24 and 48 h. Luciferase activity was normalized by β-galactosidase activity. ( f , g ) qRT–PCR analyses of the expression of AURKA and PLK1 in cells treated with CytoD or LIMKi3 for 24 and 48 h. GAPDH was used as a normalization control. ( h , i ) qRT–PCR analyses of the expression of AURKA and PLK1 in cells transfected with the indicated siRNAs for 60 h. All scale bars are 20 μm. All error bars are s.d. ( n =3 independent experiments). The P -values were determined by unpaired Student’s t -test; * P <0.05, ** P <0.01. Full size image We also investigated the time course of ciliogenesis, YAP/TAZ redistribution and cell cycle exit in response to LIMKi3 treatment ( Supplementary Fig. 8a ). There was a small decrease in the number of nuclear YAP/TAZ- and Ki67-positive cells, and the majority of cells lacked cilia until 12 h post-treatment. Thereafter, the number of ciliated cells increased, whereas Ki67-positive cells decreased continuously. Cells exhibiting nuclear YAP/TAZ also decreased consistently during the first 24 h after treatment. Unexpectedly, at 48 h post-treatment, nuclear YAP/TAZ exhibited a rebound increase unlike Ki67. CytoD treatment for 48 h also showed a similar reentry of YAP/TAZ to the nucleus in quiescent cells ( Supplementary Fig. 8b ). In accordance with these observations, our western blot analysis showed that phospho-YAP level was highest at 12 h post-treatment, whereas nuclear YAP/TAZ levels were lowest at the same time point. In addition, an increase in nuclear TAZ levels was apparent from 24 h post-treatment ( Supplementary Fig. 8c ). However, YAP/TAZ activity appears to be insufficient to elicit biological responses at 48 h post-treatment in that cells remain quiescent and exhibit lower levels of 8xGTIIC luciferase activities relative to control ( Fig. 7e ). There are several transcriptional regulators that are known to co-occupy gene promoters with YAP/TAZ [39] . Thus, it is possible that prolonged cell cycle quiescence in RPE1 cells may shift gene expression profiles, downregulating the expression of other transcriptional regulators, which support YAP/TAZ activity. To confirm that LIMK2 and TESK1 exert influence on ciliogenesis by affecting the expression of AURKA and PLK1 , we examined the expression levels of the two genes using qRT–PCR. Treatment of either CytoD or LIMKi3 decreased the levels of AURKA and PLK1 and the effect was more profound at 48 h post-treatment ( Fig. 7f,g ). Moreover, the expression levels of AURKA and PLK1 also decreased significantly in response to LIMK2 or TESK1 knockdown ( Fig. 7h,i ). These results indicate that LIMK2/TESK1 suppress ciliogenesis by upregulating the expression of YAP/TAZ target genes. LIMK2 and TESK1 affect ciliary vesicle trafficking We wondered whether YAP/TAZ are fully responsible for delimitating cellular ciliogenic activities at the downstream of LIMK2 and TESK1. If this was the case, depletion of YAP/TAZ should fully rescue the suppression of ciliogenesis observed in cells transfected with CFL1 siRNAs. As shown in Fig. 8a , combined depletion of CFL1 and YAP/TAZ resulted in only partial rescue of the inhibitory effect of CFL1 knockdown on serum starvation-mediated ciliogenesis. This suggests that YAP/TAZ are not the only downstream effectors of the actin cytoskeleton remodelling that regulates ciliogenesis. Consistent with this possibility, YAP/TAZ knockdown did not fully recapitulate the effect of CytoD on cilium assembly: cilia formed by CytoD treatment were significantly longer ( Fig. 8b ). The perturbation of actin cytoskeleton dynamics has been reported to facilitate centrosomal accumulations of the vesicles carrying ciliary cargo (ciliary vesicles) during ciliogenesis [13] , [15] . Thus, we examined whether trafficking of ciliary vesicles is affected by either LIMK2 or TESK1 knockdown. To capture vesicle trafficking activities at the initiation stages of ciliogenesis, we arrested the progression of ciliogenesis using CEP164 knockdown [40] and visualized ciliary vesicles in RPE1-Smo-EGFP cells. In this condition, depletion of either LIMK2 or TESK1 promoted the accumulation of Smo-EGFP/RAB11-positive vesicles to the pericentrosomal area ( Fig. 8c,d ), indicating that LIMK2/TESK1 plays a role in suppressing the directional trafficking of ciliary vesicles to the ciliary base. Then we examined the localization of LIMK2 and TESK1. As shown in Fig. 8e , a pool of LIMK2 and TESK1 localized to the centrosome. These data suggest that functions of LIMK2 and TESK1 in ciliogenesis control include the modulation of directional trafficking of ciliary vesicles in addition to YAP/TAZ regulation. 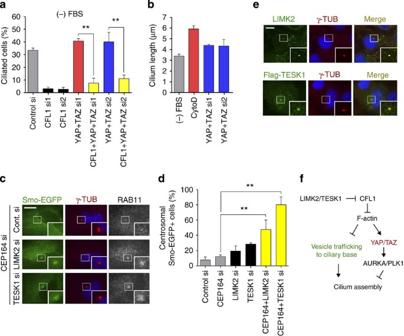Figure 8: LIMK2 and TESK1 control vesicle trafficking to the pericentrosomal area. (a) Quantification of ciliogenesis in RPE1 cells transfected with the indicated siRNAs for 60 h. Cells were serum-starved for final 24 h. (b) Graph showing the measurement of ciliary length in cells treated with serum starvation (24 h), CytoD (24 h) or YAP/TAZ mix siRNAs (60 h). (c) Immunofluorescence images showing the effect of LIMK2 and TESK1 knockdown on the trafficking of tentative ciliary vesicles double-positive for Smo-EGFP and endogenous RAB11. CEP164 was also depleted to arrest ciliogenesis at the initiation stage of ciliogenesis. Insets are magnified view of the centrosomal area. (d) Quantification of experiments illustrated inc. (e) Subcellular localization of endogenous LIMK2 and flag-tagged TESK1, which was transiently expressed. Insets are magnified view of the centrosomal area. (f) A proposed model for the regulation of cilium assembly by actin-dependent pathways. All scale bars are 10 μm. All error bars are s.d. (n=3 independent experiments). TheP-values were determined by unpaired Student’st-test; **P<0.01. Figure 8: LIMK2 and TESK1 control vesicle trafficking to the pericentrosomal area. ( a ) Quantification of ciliogenesis in RPE1 cells transfected with the indicated siRNAs for 60 h. Cells were serum-starved for final 24 h. ( b ) Graph showing the measurement of ciliary length in cells treated with serum starvation (24 h), CytoD (24 h) or YAP/TAZ mix siRNAs (60 h). ( c ) Immunofluorescence images showing the effect of LIMK2 and TESK1 knockdown on the trafficking of tentative ciliary vesicles double-positive for Smo-EGFP and endogenous RAB11. CEP164 was also depleted to arrest ciliogenesis at the initiation stage of ciliogenesis. Insets are magnified view of the centrosomal area. ( d ) Quantification of experiments illustrated in c . ( e ) Subcellular localization of endogenous LIMK2 and flag-tagged TESK1, which was transiently expressed. Insets are magnified view of the centrosomal area. ( f ) A proposed model for the regulation of cilium assembly by actin-dependent pathways. All scale bars are 10 μm. All error bars are s.d. ( n =3 independent experiments). The P -values were determined by unpaired Student’s t -test; ** P <0.01. Full size image Emerging lines of evidence have shown that dynamic remodelling of actin filament networks provides critical cues for the regulation of ciliogenesis and cilium length. Here, we provide evidence for the role of YAP/TAZ and vesicle trafficking in ciliogenesis control as downstream elements of actin remodelling. This conclusion is based on the following findings. First, cytoplasmic retention of YAP/TAZ, which was promoted either by high cell density or CytoD treatment, correlated with the induction of ciliogenesis. Second, depletion of YAP/TAZ caused a significant increase in the number of ciliated cells in the absence of other ciliogenic stimulations. Conversely, hyperactivation of YAP/TAZ suppressed serum starvation-mediated ciliogenesis. We also found that actin remodelling factors LIMK2 and TESK1 suppress ciliogenesis by regulating the expression of YAP/TAZ target genes and the directional trafficking of ciliary vesicles to ciliary base. Taken together, these results lead us to propose a model in which actin cytoskeletal remodelling controls ciliogenesis through the orchestration of intracellular trafficking and transcriptional programme. YAP/TAZ activity is regulated by mechanical/physical stimuli exerted by the cell’s morphology, contracture or extracellular matrix rigidity [19] . Recent studies have shown that actin stress fibre can regulate YAP/TAZ through the Hippo pathway effectors LATS1/2 (refs 27 , 28 ). Interestingly, the actin cytoskeleton can also directly regulate YAP/TAZ activity independent of the Hippo pathway [21] . F-Actin-capping/severing proteins CFL, CapZ and Gelsolin appear to play key roles in suppressing YAP/TAZ activity [20] . Among them, CFL facilitates actin dynamics by promoting cleavage and depolymerization of actin filaments [37] , and is negatively regulated by Rho-ROCK signalling [41] . Here we show that a ROCK inhibitor facilitates ciliogenesis, supporting inhibitory roles of YAP/TAZ in ciliogenesis. Furthermore, we identify LIMK2 and TESK1, upstream inhibitory kinases of CFL, as potent negative regulators of ciliogenesis. The fact that depletion of LATS1/2 does not inhibit serum starvation-mediated ciliogenesis suggests that actin-dependent molecules other than LATS1/2 play a major role in suppressing YAP/TAZ during ciliogenesis. However, our results do not exclude the involvement of the Hippo pathway in ciliogenesis control. Indeed, a recent paper showed that the MST1/2-SAV1 complex of the Hippo pathway promotes ciliogenesis by dissociating the AURKA/HDAC6 cilium-disassembly complex [24] . Therefore, it appears that Hippo-YAP pathway components and ciliogenesis regulators functionally interact at multiple levels, highlighting the importance and complexity of the association. Although actin destabilization induces the formation of primary cilia in vitro , positive roles of F-actin networks in ciliogenesis have been also proposed in different contexts. In multiciliated cells, the apical web-like actin enrichment is essential for the docking of basal bodies, which are produced by de novo assembly within the cytoplasm [42] , [43] . Apical actin enrichment appears to be mediated by RhoA activity in airway epithelial cells [42] , and the planar cell polarity pathway governs the activation of RhoA at the basal bodies [44] . It is also noteworthy that the assembly of primary cilia also requires the migration of the centriole/basal body to the apical plasma membrane, which involves actin-myosin-based mechanisms. Moreover, Meckel–Gruber syndrome protein Meckelin functions with an actin-binding protein filamin A, and loss-of-function mutations in Meckelin cause defects in centriole migration, which interfere with ciliogenesis [45] . Thus, the completion of multiple steps of ciliogenesis may require successive remodelling of actin cytoskeleton architecture. TAZ knockout mice present with multiple renal cysts that lead to severe polycystic kidney disease [46] , [47] , [48] . TAZ localizes to primary cilia in mouse BMK cells [48] , and cilia in mouse IMCD cells depleted of TAZ are short and exhibit apparent structural defects [46] . Loss of TAZ has been shown to cause abnormal accumulation of polycystin 2 (PC2), a Ca 2+ -permeable cation channel, whose dysfunction has been implicated in cyst development [48] , [49] , although how elevation of PC2 levels interferes with cilium assembly remains unclear. It is noteworthy that a Pkd2 mutant mouse in which PC2 levels are substantially decreased also displays defective ciliogenesis [50] . In addition, NIMA-related kinase 1 (NEK1) was shown to interact with TAZ and maintain normal levels of PC2 (ref. 49 ). Interestingly, NEK1 can suppress cilium assembly [51] , [52] , while a RNAi library screen identified NEK1 as a positive ciliogenesis regulator [53] . Apparent loss-of-function mutations of NEK1 in human cause ciliopathy-like phenotypes [54] . Although the involvement of NEK1 in the regulation of ciliogenesis is obvious, it is not clear whether NEK1 is positive or negative regulator. Similarly, TAZ knockout mice show defective cilia, whereas we found that TAZ depletion is sufficient to induce ciliogenesis at least in RPE1 cells. Thus, the exact roles of TAZ in ciliogenesis control might be cell type-specific. Alternatively, it is plausible that TAZ loss-of-function may cause an abnormal or premature elevation of ciliogenic activity, which interferes with normal cellular differentiation of renal progenitor cells and eventually causes kidney cysts with defective cilia. Ciliogenesis is generally considered as linked to quiescent (G0) phase of the cell cycle in cultured mammalian cells [7] . Indeed, enhanced ciliogenic activity in cells treated with CytoD or in cells depleted of LIMK2/TESK1 was accompanied by cell cycle exit, suggesting that the actin cytoskeleton can affect ciliogenesis through its impact on cell proliferation ( Supplementary Figs 2a and 7c ). However, CytoD treatment and LIMK2/TEKS1 knockdown induced ciliogenesis even in cells arrested in early S phase. Moreover, ciliogenesis occurs in actively cycling cells during embryonic development [10] . Thus, ciliogenesis can be uncoupled from cell cycle exit. The coincidence of cell cycle exit and ciliogenesis in cultured cells might be ascribed to the dual roles of YAP/TAZ: promotion of cell proliferation and suppression of ciliogenesis. Thus, it might be natural that actin cytoskeletal remodelling that controls YAP/TAZ activity simultaneously affect both cell proliferation and ciliogenesis. Interestingly, contact-mediated inhibition of cell proliferation is apparently absent in actively proliferating early embryos. It is tempting to speculate that this temporal uncoupling of cell density and cell proliferation might explain how embryonic cells can support ciliogenesis even when cells are actively cycling. Previous studies have reported that inhibition of F-actin assembly either by application of CytoD or depletion of ARP2/3 complex subunits using siRNAs or miRNA mir-129-3p promote pericentrosomal accumulations of ciliary vesicles positive for recycling endosome markers [13] , [15] . Accordingly, we observed that actin architecture remodelling induced by LIMK2 and TESK1 knockdown facilitates the directional trafficking of Smo-EGFP/RAB11-positive vesicles to the pericentrosomal area. In addition, the inhibitory effect of CFL knockdown on ciliogenesis in the cells co-depleted with YAP/TAZ was rescued only partially, which suggesting that directional trafficking of ciliary vesicles also plays a pivotal role in addition to YAP/TAZ activity in ciliogenesis. The actin cytoskeleton is known to play key roles in endocytosis and exocytosis, providing filament networks and bundles to facilitate membrane remodelling/sorting and vesicle movement [41] , [55] . Actin destabilization causes discernible morphological changes in various membrane organelles and interferes with regular endosomal trafficking [56] . Interestingly, CytoD treatment enhances the formation of RAB8-positive membrane tubules, presumably by disrupting the route of recycling endosomes [57] . We can envision that actin cytoskeleton remodelling can modulate potential competition between endocytic recycling route and the membrane trafficking route supporting ciliogenesis and ciliary membrane elongation. However, understanding the exact mechanisms underlying the link between actin dynamics and ciliary vesicle trafficking requires further investigation. In summary, we propose that actin dynamics may control cellular ciliogenic activity by orchestrating bifurcated molecular pathways. First, an increase in actin dynamics rapidly reorganizes intracellular membrane transport, stimulating the trafficking pathway to the pericentrosomal area, which delivers vesicles destined for cilia. Second, elevated actin dynamics or actin destabilization impacts on the YAP/TAZ pathway, which might be a key component of transcriptional networks governing ciliogenesis and cell proliferation. Our work provides new insights into how cells sense mechanical stimuli and transduce the information into ciliogenesis control. Cell culture RPE1 cells were cultured in DMEM/F12 (Welgene) supplemented with 10% FBS and 1% penicillin/streptomycin. RPE1-Smo-EGFP cells were established as previously reported [13] . HEK293T cells were cultured in DMEM (Welgene) supplemented with 10% FBS and 1% penicillin/streptomycin. A549 cells were cultured in RPMI1640 (Welgene) supplemented with 10% FBS and 1% penicillin/streptomycin. RPE1 and HEK293T cells were purchased from American Type Culture Collection, and A549 cells were provided by Professor Tae-Young Yoon (KAIST). siRNA and plasmid transfection siRNA transfection was performed with Lipofectamine RNAiMAX (Invitrogen) according to the manufacturer’s reverse transfection protocol. Cells were fixed 48–72 h after transfection. Dharmacon ON-TARGETplus siRNA SMARTpools (GE Healthcare Life) were used for screening actin regulatory kinases ( Fig. 6a ). The sequences of other siRNAs used in this study are provided in Supplementary Table 1 . Plasmid transfection was performed with Lipofectamine LTX and PLUS reagent (Invitrogen) according to the manufacturer’s forward transfection protocol. Cells were fixed 24–36 h after transfection. To induce serum starvation-mediated ciliogenesis, cells were incubated in serum-free media for 24 or 48 h before fixation. Plasmids and reagents Human TESK1 cDNA was provided by Addgene (Plasmid #20650), and subcloned into the flag-tagged pcDNA3.1 (+) vector (Life Technologies). EGFP-tagged human RAB11 was provided by Addgene (Plasmid #12674), and EGFP-tagged human RAB8 was also provided by Addgene (Plasmid # 31735). Raichu-RhoA [58] was kindly donated by Professor Michiyuki Matsuda (Kyoto University). 8xGTIIC-luciferase cDNA was provided by Addgene (Plasmid #34615) [21] . β-Galactosidase control vector, pcDNA3.1-His-lacZ was purchased from Invitrogen. CytoD (Sigma-Aldrich) was treated at 200 nM for the indicated times. CHX (Sigma-Aldrich) was added at 20 μg ml −1 24 h before fixation. Thymidine (Sigma-Aldrich) was treated at 2 mM 36 h before fixation to arrest cells in early S phase. LPA (Sigma-Aldrich) was added at 1–30 μM 24 h before fixation. LIMKi3 (Merck Millipore) was treated at 1–20 μM for the indicated times. Retroviral infection To produce retroviral particles, HEK293T cells were transfected with pMSCV-puro (empty vector), pMSCV-puro-YAP-5SA or pMSCV-puro-YAP-5SA-S94A constructs (provided by Professor Dae-Sik Lim, KAIST) with Lipofectamine LTX and PLUS reagent according to the manufacturer’s forward transfection protocol. These constructs were co-transfected with retroviral packaging plasmids, pCMV-Gag-Pol and pCMV-VSV-G (provided by Professor Dae-Sik Lim, KAIST). Forty-eight hours after transfection, retroviral supernatant was supplemented with 4 μg ml −1 of polybrene, filtered through a 0.45-μm filter, and used to infect RPE1 cells. Thirty-six hours after infection, cells were selected with 8 μg ml −1 puromycin (Sigma-Aldrich) in culture medium for 24 h. To induce serum starvation-mediated ciliogenesis, cells were incubated in serum-free medium for 48 h before fixation. Irradiation and cell cycle analysis RPE1 cell were treated with ionizing radiation at a dose of 5 Gy min −1 using a Cs-137 irradiator (Gammacell 3000, Best Theratronics) for 90 s to arrest cells in G2/M phase. DNA content was analysed with BD FACSCalibur flow cytometer (BD Biosciences). The percentage of cells in G1, S and G2 phases was determined using FlowJo software (Tree Star). Immunofluorescence For indirect immunofluorescence, cells were grown in 8-well Lab-Tek II chamber slides (Nunc) or 96-well plates (BD Falcon or ibidi) for the indicated times and fixed in methanol for 2 min at −20 °C or in 4% paraformaldehyde for 7 min at room temperature (RT; for YAP/TAZ and Phalloidin staining). Paraformaldehyde fixation was followed by 5 min permeabilization step in 0.1% Triton X-100 (Sigma-Aldrich). After blocking with 5% FBS for 10 min, cells were incubated with primary antibodies at RT for 1 h. Primary antibodies were detected with Alexa Fluor 488-, 594- or 647-conjugated secondary antibodies (Life Technologies) for 1 h at RT. For F-actin staining, cells were labelled with Alexa Fluor 594-Phalloidin (Life Technologies) as described by the manufacturer’s protocol. Cells were mounted with mounting solution (75% glycerol, 20 nM Tris (pH 8.8), and 0.02% NaN 3 ) containing 0.5 μg ml −1 4,6-diamidino-2-phenylindole (Sigma-Aldrich) for fluorescence microscope imaging or Dako fluorescent mounting medium (Dako) for confocal microscope imaging. All primary antibodies used in this study are described in Supplementary Table 2 . Fluorescence microscopy Immunofluorescence images were acquired using a DeltaVision Spectris Imaging System (Applied Precision) equipped with an Olympus IX70 inverted microscope, × 20 objective lens (0.4 numerical aperture (NA), Plan-Achromat), × 60 oil-immersion objective lens (1.42 NA, Plan-Achromat), a CoolSNAP HQ2 CCD camera (Photometrics), and SoftWorx software (Applied Precision). Fields were selected randomly for each well on the basis of the number of 4,6-diamidino-2-phenylindole-stained nuclei in order to exclude bias from the differences in cell density. Z-stack imaging was performed using a Zeiss LSM 780 confocal laser scanning microscope equipped with a Zeiss Axio Observer Z1 inverted microscope, × 40 water-immersion objective lens (1.1 NA, LD C-Apochromat), × 63 oil-immersion objective lens (1.4 NA, Plan-Apochromat), 32-channel GaAsP spectral detector (Quasar) and ZEN software (Nikon). Side views shown in Supplementary Fig. 6a were acquired using XZ optical sections of Z-stack confocal microscopic images (30 planes separated by 0.2 μm interval) by using ZEN software (Nikon). The acquired images were processed and analysed using ImageJ software (NIH), and sized and placed in figures using Adobe Photoshop CS6 (Adobe Systems). Live cell imaging RPE1–Smo–EGFP cells were treated with CytoD for up to 3 h in the presence of 10% FBS. Time-lapse images of live cells were acquired using a DeltaVision Spectris Imaging System (Applied Precision) equipped with an environmental chamber. FRET imaging of RhoA activity RPE1 cells were transfected with Raichu-RhoA for 12 h before fixation. After paraformaldehyde fixation, cells were stained with YAP/TAZ antibody, and mounted with Dako fluorescent mounting medium. All images were captured by a Nikon A1R confocal laser scanning microscope equipped with a Nikon Eclipse Ti-E inverted microscope, × 60 oil-immersion objective lens (1.4 NA, CFI Plan-Apochromat), 4-channel PMT detector (Nikon) and Nikon imaging software (NIS-element AR, Laboratory Imaging). Emission ratio imaging was performed with a 457-nm excitation laser/535 nm emission YFP HYQ filter (Nikon). After background subtraction, ratio images of FRET/CFP were created and analysed with Nikon imaging software (NIS-element AR, Laboratory Imaging) to represent FRET efficiency. Western blotting For western blot analysis, cells were lysed on ice in RIPA lysis buffer (20 mM HEPES (pH 7.5), 150 mM NaCl, 1% NP-40, 0.25% sodium deoxycholate and 10% glycerol) supplemented with protease and phosphatase inhibitors (Merck Millipore). Cell lysates were sonicated with a Branson Digital Sonifier 250 (Branson Ultrasonics) and then subjected to centrifugation for 10 min at 4 °C, 13,000 r.p.m. (18,400 r.c.f.). Protein concentrations of the supernatants were quantitated through the detergent-insensitive Pierce BCA protein assay kit (Thermo Scientific). Total protein lysates were added with Lamni buffer (62.5 mM Tris, 2% SDS, 5% 2-mercaptoethanol, 10% glycerol and 0.02% bromophenol blue) and denatured at 95 °C for 5 min. Aliquots of each protein lysate (10–20 μg) were subjected to SDS–polyacrylamide gel electrophoresis for 90–100 min in 100 V. After electrophoresis, proteins were transferred to nitrocellulose membranes for 80 min in 300 mA, and blocked for 30 min with blocking solution (TBST buffer with 5% skim milk and 0.02% NaN 3 ). Primary antibodies were incubated for overnight at 4 °C ( Supplementary Table 2 ). Incubation with secondary peroxidase-coupled antibody (Santa Cruz Biotechnology) was performed for 1 h at 4 °C. Antibodies targeted proteins were visualized by using the enhanced chemiluminescence (ECL) western blot detection solution (Neuronex and LumiGLO). The full blots of the cropped images are presented in Supplementary Fig. 9 . Subcellular fractionation Nuclear and non-nuclear fractions were prepared from RPE1 cells using the NE-PER nuclear and cytoplasmic extraction reagent (Thermo Scientific) according to the manufacturer’s instructions except a cell harvesting procedure, which was done by using a cell scraper other than trypsin-EDTA because the change of cell morphologies by trypsinization can affect the localization of YAP/TAZ. Luciferase assay For luciferase assay, cells were plated on 96-well plates and transfected when 50–60% confluency with YAP/TAZ-responsive reporter, 8xGTIIC-luciferase and β-galactosidase control vector, pcDNA3.1-His-lacZ with Lipofectamine LTX and PLUS reagent according to the manufacturer’s forward transfection protocol. Cells were harvested with reporter lysis buffer after 12 h and luciferase assays were performed with luciferase assay system (Promega) according to the manufacturer’s instruction. β-Galactosidase activity was measured using a β-Galactosidase enzyme assay system (Promega) and was used to normalize the luciferase activity for transfection efficiency. RNA extraction and qRT–PCR Total RNA was extracted from the samples using the RNeasy kit (Qiagen) according the manufacturer’s instructions. Trace of DNA was removed using a RQ1 RNase-Free DNase (Promega), and 1 μg of total RNA was reverse transcribed into cDNA using M-MLV reverse transcriptase (Promega). qRT–PCR was performed using iQ SYBR Green Supermix (Bio-Rad) with primers spanning two or more exons and optimized for real-time PCR. The primers were designed using Primer-BLAST [59] except for those of AURKA, which were obtained from AccuTarget real-time PCR primer library (Bioneer). The sequences for all primers used in this study are provided in Supplementary Table 3 . qRT–PCR was performed using CFX96 real-time PCR detection system (Bio-Rad). Reaction specificity was confirmed by melting curve analysis. Relative gene expression was analysed by comparative Ct method [60] using the CFX Manager software (Bio-Rad). Quantification and statistical analysis Primary cilia were stained with antibody specific for poly-glutamylated Tubulin (glu-TUB) or ARL13B. To acquire the percentage of ciliated cells, only cilia whose length are longer than 1.0 μm were quantified manually (see also Supplementary Fig. 1a ), and cell count was performed automatically by using CellProfiler software (Broad Institute) [61] . At least, 100–150 cells were counted in each experiment. The length of cilia and western blot band intensity was measured by using ImageJ software (NIH). The quantification of YAP/TAZ localization was performed automatically by using a custom-made pipeline of CellProfiler software (Broad Institute; see also Supplementary Fig. 3c ). The statistical data were obtained from at least two independent experiments performed in duplicate. The data of qRT–PCR and luciferase assay were normalized by dividing all values of control and treatment by the mean of the control [62] . The differences between experimental values were considered significant when P -value was <0.05 in an unpaired Student’s t -test using GraphPad Prism 5.0 (GraphPad Software). How to cite this article: Kim, J. et al. Actin remodelling factors control ciliogenesis by regulating YAP/TAZ activity and vesicle trafficking. Nat. Commun. 6:6781 doi: 10.1038/ncomms7781 (2015).